Structural correlations in the generation of polaron pairs in low-bandgap polymers for photovoltaics Polymeric semiconductors are materials where unique optical and electronic properties often originate from a tailored chemical structure. This allows for synthesizing conjugated macromolecules with ad hoc functionalities for organic electronics. In photovoltaics, donor–acceptor co-polymers, with moieties of different electron affinity alternating on the chain, have attracted considerable interest. The low bandgap offers optimal light-harvesting characteristics and has inspired work towards record power conversion efficiencies. Here we show for the first time how the chemical structure of donor and acceptor moieties controls the photogeneration of polaron pairs. We show that co-polymers with strong acceptors show large yields of polaron pair formation up to 24% of the initial photoexcitations as compared with a homopolymer ( η =8%). π-conjugated spacers, separating the donor and acceptor centre of masses, have the beneficial role of increasing the recombination time. The results provide useful input into the understanding of polaron pair photogeneration in low-bandgap co-polymers for photovoltaics. Organic photovoltaics are an emerging technology based on molecular materials, which is expected to have an important role in the field of devices for renewable energy. The most promising material systems are thin films made of blends between a conjugated polymer and a suitable electron-acceptor molecule, typically a fullerene derivative. The primary steps in photovoltaic action are the absorption of light in correlation to π–π* transitions by the conjugated molecule and charge separation at the heterojunction with the fullerene. While the power conversion efficiency has been demonstrated to depend on a number of different factors, such as morphology of the blend-film [1] , carrier mobility [2] and device architecture [3] , the first fundamental processes remain photon absorption by a chromophore and the dissociation of the resulting electron-hole pair. Light absorption by the polymer has been largely improved towards the near infrared (NIR) spectral region by the introduction of low-bandgap co-polymers [4] , [5] . Exciton dissociation, however, remains to be understood and has recently been the subject of several investigations [6] , [7] , [8] , [9] , [10] . The basic model considers light absorption generating strongly bound Frenkel excitons (binding energy>0.5 eV), which then dissociate primarily at the interface with the fullerene [11] . There, the large energy offset (≥0.5 eV) between the lowest unoccupied molecular orbitals (LUMOs) of polymer and fullerene, possibly gated by the formation of hot delocalized states [9] , drives exciton dissociation and charge separation. This is supposed to occur only after diffusion of the excitons in the polymer, which is usually forming an interpenetrating network of domains with the fullerene [12] . However, several experimental and theoretical studies have suggested that the primary photoexcitations in pristine conjugated polymers are not only excitons but also polaron pairs, the latter being more separated electrons and holes with a weaker Coulomb attraction [13] , [14] , [15] . Very recently, it has been reported that polaron pairs, formed within the polymer domains, have a significant role in photovoltaic action and are envisaged to be as important as excitons, provided their yield is substantial [16] , [17] , [18] . Although revealing important phenomena for the functioning of solar cells, these and other optical investigations have focussed on the dynamics of excitons [19] or charge-separated states when the polymer is mixed with the fullerene [20] , [21] , [22] . The question, of what the polaron pair generation yield in pristine donor–acceptor co-polymers actually is, remains largely unanswered while being of very large relevance for understanding and improving photovoltaics. For example, discrepancies between theoretically predicted solar cell efficiencies, based on Onsager–Braun models, and the higher measured values may originate from the previously disregarded contribution of polaron pairs forming directly in the polymer [2] , [7] . In these low-bandgap macromolecules, electron donating and accepting moieties are copolymerized and form the repeat unit of the polymeric chain. The two moieties are conjugated and form a ladder of energy levels typically exhibiting a smaller energy gap between the frontier orbitals, highest occupied molecular orbital (HOMO) and LUMO, than the isolated uncoupled donor and acceptor. This concept is schematically illustrated in Fig. 1a . Optical transitions between the frontier orbitals are responsible for the absorption extending in the NIR. Such unique optical properties can hardly be achieved with conjugated homopolymers. Thus, for homopolymers power conversion efficiencies above 6% are scarce [23] , and likely limited by a poor overlap with the solar spectrum in the NIR. Although the improved light harvesting characteristics of donor–acceptor co-polymers have been often attributed to the low bandgap, it remains a crucial question to correlate the nature of the primary photoexcitations with the molecular design. In particular, how the structure of the alternating donors and acceptors may favour the generation of polaron pairs, for example, by localization of the electron and hole on the accepting and donating segment, respectively. Answering this question is of relevance, as in polaron pair states, electrons and holes have weaker binding than in excitonic configurations. Therefore, their separation might require less pronounced offsets in heterojunctions and thus a decreased energy and voltage loss for complete charge separation in solar cells [24] , [25] . 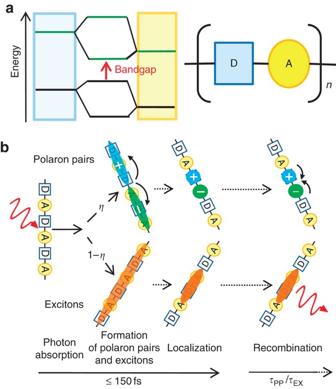Figure 1: Electronic structure and photoinduced polaron pairs in co-polymers. (a) Simplified electronic structure of donor–acceptor low-bandgap co-polymers with HOMO and LUMO levels of the two moieties coupling to form the energy levels of the polymeric chain. (b) Illustration of the photoinduced processes in co-polymers; on light absorption a delocalized exciton or a polaron pair is formed with a yieldη, this occurs within the first 150 fs. The polaron pairs decay by recombination on a longer time scale. D and A indicate donor and acceptor moieties. Figure 1: Electronic structure and photoinduced polaron pairs in co-polymers. ( a ) Simplified electronic structure of donor–acceptor low-bandgap co-polymers with HOMO and LUMO levels of the two moieties coupling to form the energy levels of the polymeric chain. ( b ) Illustration of the photoinduced processes in co-polymers; on light absorption a delocalized exciton or a polaron pair is formed with a yield η , this occurs within the first 150 fs. The polaron pairs decay by recombination on a longer time scale. D and A indicate donor and acceptor moieties. Full size image Here, we employ time-resolved photoinduced absorption spectroscopy to probe the generation and recombination of polaron pairs in a series of model donor–acceptor co-polymers of interest for photovoltaic devices. In particular, we address the role of acceptor strength or difference in electron affinity and donor–acceptor topology within the chain in controlling the photoinduced dynamics of polaron pairs. Figure 1b illustrates the conceptual question to be addressed in the experiments: what is the yield ( η ) of polaron pair formation from the initial overall amount of photoexcitations? In addition, what are the recombination dynamics for the two populations of excitons and polaron pairs? NIR pump probe spectroscopy offers a formidable experimental tool to pinpoint polaron pairs and watch their evolution in real time. Having at hand a unique series of materials with systematic variations to the chemical structure, we show how changing the alternation length and electron affinity imbalance has a strong influence on the generation yield and the recombination dynamics. The experimental results for the co-polymers are compared with the model system regioregular poly(3-hexylthiophene) (P3HT), which is one of the most studied homopolymers in solar cells [26] . All co-polymers exhibit significantly larger polaron pair yields compared with P3HT, while exhibiting recombination dynamics, which are fundamentally correlated to their chemical structure. The results unravel important aspects on the role of chemical structure in controlling the primary photoexcitations in conjugated co-polymers. Low-bandgap co-polymers We focussed our attention on four different co-polymers having the same 4,4′- bis -(2-ethylhexyl)- 4H -cyclopenta[2,1- b ;3,4- b ′]-dithiophene donor moiety indicated as CPDT and different acceptors; benzo-[1,2- c ;4,5-c′] bis [1,2,5]thiadiazole] (BDT), (2,1,3-benzothiadiazole) (BT) 2,3-diphenyl-5,7- bis (2-thienyl)thieno[3,4- b ]pyrazine (2TTP) and -4,7- bis (2-thienyl)-2,1,3-benzothiadiazole (2TBT). The chemical structures of the respective compounds are reported in Fig. 2a–d and details about their synthesis outlined in the Methods section. The four donor–acceptor co-polymers can be divided into two categories. To the first category belong PCPDT-BDT and PCPDT-BT ( Fig. 2a,b ); they are both based on benzothiadiazole-like acceptors, that are directly linked to the CPDT donor. They differ in the electronegativity of the isolated acceptor, which is larger for BDT (−3.21 eV) than for BT (−1.81 eV) [27] . The second category has different acceptors as well, but the two co-polymers share an on-chain topology that is different compared with one of the first. Here, the CPDT donor is linked to the acceptor via thiophene spacers. We refer to them as spacers in the sense that they further separate the donor and acceptor centres of mass and are chemically similar to the CPDT donor. Among PCPDT-2TBT and PCPDT-2TTP, the latter is expected to have the acceptor with the higher electron affinity as confirmed below. 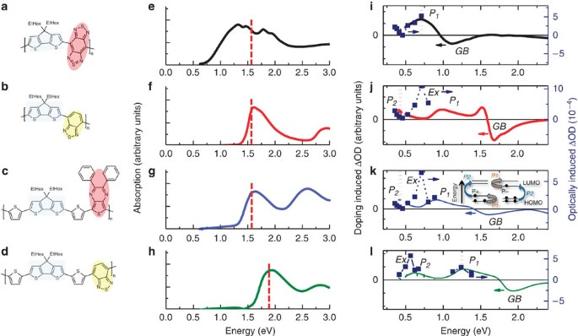Figure 2: Excitons and polaron pairs spectra of low-bandgap co-polymers. Chemical structure of the repeat unit for the co-polymers: (a) PCPDT-BDT, (b) PCPDT-BT, (c) PCPDT-2TTP and (d) PCPDT-2TBT. The donor and acceptor moieties are indicated with grey and yellow/red shaded areas, respectively. Red shaded areas indicate acceptor moieties with larger electron affinities. Absorption spectra of: (e) PCPDT-BDT, (f) PCPDT-BT, (g) PCPDT-2TTP and (h) PCPDT-2TBT. The vertical dashed lines indicate the pump photon energies for the transient absorption experiments. (i) PCPDT-BDT, (j) PCPDT-BT, (k) PCPDT-2TTP, (l) PCPDT-2TBT doping-induced ΔOD spectra as solid lines obtained by adding SbCl5to the respective polymer solutions.GBindicates ground-state bleaching,P1first polaron band,Exexciton absorption band,P2second polaron band. The blue squares show the transient absorption spectra recorded at zero time delay between the pump and probe beam. The respective pump beam wavelengths are indicated on the corresponding linear absorption graphs. The vertical dashed red lines indicate the choice of probe photon energies for determining the polaron pair yields in the experiments ofFig. 5. The inset in (k) sketches theP1andP2polaron transitions. Figure 2: Excitons and polaron pairs spectra of low-bandgap co-polymers. Chemical structure of the repeat unit for the co-polymers: ( a ) PCPDT-BDT, ( b ) PCPDT-BT, ( c ) PCPDT-2TTP and ( d ) PCPDT-2TBT. The donor and acceptor moieties are indicated with grey and yellow/red shaded areas, respectively. Red shaded areas indicate acceptor moieties with larger electron affinities. Absorption spectra of: ( e ) PCPDT-BDT, ( f ) PCPDT-BT, ( g ) PCPDT-2TTP and ( h ) PCPDT-2TBT. The vertical dashed lines indicate the pump photon energies for the transient absorption experiments. ( i ) PCPDT-BDT, ( j ) PCPDT-BT, ( k ) PCPDT-2TTP, ( l ) PCPDT-2TBT doping-induced ΔOD spectra as solid lines obtained by adding SbCl 5 to the respective polymer solutions. GB indicates ground-state bleaching, P 1 first polaron band, Ex exciton absorption band, P 2 second polaron band. The blue squares show the transient absorption spectra recorded at zero time delay between the pump and probe beam. The respective pump beam wavelengths are indicated on the corresponding linear absorption graphs. The vertical dashed red lines indicate the choice of probe photon energies for determining the polaron pair yields in the experiments of Fig. 5 . The inset in ( k ) sketches the P 1 and P 2 polaron transitions. Full size image Ground- and excited-state absorption Figure 2e–h shows the absorption spectra of the different compounds deposited as thin films. All conjugated co-polymers have an absorption onset extending in the NIR region of the spectrum (<1.7 eV), exhibiting slightly different bandgaps. As for other very similar co-polymers [28] , the energetic position of the first absorption band (S 1 ) is mainly determined by the HOMO donor –LUMO acceptor energy difference and the electronic coupling between them as schematically shown in Fig. 1a (ref. 29 ). PCPDT-BDT having the most electronegative acceptor moiety among the materials presented here, shows an absorption onset starting at a photon energy ~0.8 eV ( Fig. 2e ). PCPDT-BT and PCPDT-2TBT have the same acceptor, but the presence of the thiophene spacers in PCPDT-2TBT, further separates the mass centres of the donating and accepting moieties, likely influencing the electronic structure of the coupled system. This results in a slightly blue-shifted absorption onset of PCPDT-2TBT ( Fig. 2h ) with respect to PCPDT-BT ( Fig. 2f ). In PCPDT-2TTP ( Fig. 2g ), the two thiophene spacers decreasing the coupling are present, but the stronger acceptor characteristics of TP with respect to BT appear in an S 0 -S 1 absorption band located at a smaller photon energy with respect to the other copolymer with spacers, PCPDT-2TBT. Optical signatures of polarons are evident in the infrared and originate from the bandgap renormalization on removal of charge neutrality on the π-conjugated system [30] , [31] . We have determined the energetic position of the polaron absorption bands in the infrared by chemical doping with the oxidizing dopant SbCl 5 and quantum-chemical calculations [32] , [33] . SbCl 5 is known to be a strong oxidizing agent and to generate a hole-polaron in the ground state of most conjugated polymers [34] , [35] . Figure 2i–l shows the corresponding dopant induced variation in the optical density spectra (solid curves), measured by adding a small amount of SbCl 5 (4% weight) to the respective polymers. The differential spectra (ΔOD), obtained by subtraction of the spectrum of the undoped sample from the doped one, reveal prominent bands in the infrared spectral region. A recurrent feature in the spectra is the presence of two absorption bands P 1 and P 2 , which in the simplest picture are assigned to the interband (polaron→LUMO) and intraband (HOMO→polaron) electronic transitions, respectively. The inset of Fig. 2k illustrates these transitions and the assignment is supported by the theoretical results, though these show that considerable electronic configuration mixing occurs in these low-bandgap polymers ( Supplementary Methods and Supplementary Fig. S3 ). On the high-energy side, all the ΔOD spectra exhibit a ground-state bleaching, negative absorption change, matching the correspondent absorption profiles commented above with some differences in the onset due to electro-absorption features appearing as absorption peaks or shoulders on the blue side of the P 1 bands [36] . The short-living nature of photoinduced polaron pairs calls for spectroscopic probes on a short time scale, such as femtosecond pump-probe spectroscopy. In the same set of figures, we report the optically induced transient differential absorption (ΔOD) spectra recorded on photoexcitation in the first absorption band (S 0 →S 1 ) and probing at several photon energies in the infrared (dashed blue squares). The spectra, here shown for zero time delay between pump and probe, exhibit similarities to the dopant-induced spectra in the region of P 1 and P 2 transitions and lead us to the proposition that these are absorption bands of electron and hole polaron pairs generated on photoexcitation. Some deviations between the dopant-induced and photoinduced spectra are apparent. For example, the spectra of PCPDT-BT, -2TBT and -2TTP show an additional feature indicated as Ex. Since hole- and electron-polarons have a similar spectrum as we show below, Ex is likely corresponding to excitonic absorptions from S 1 to S n . Spectrally resolved dynamics of excitons and polaron pairs The assignment of the Ex band to excitonic species is supported by its faster dynamics with respect to the polaron pair bands. 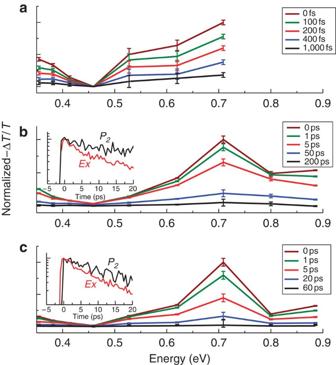Figure 3: Exciton and polaron pair dynamics. ΔT/Tspectra recorded at different pump-probe delay times for the co-polymers PCPDT-BDT (a), PCPDT-BT (b) and PCPDT-2TTP (c).P1andP2indicate the polaron transitions, whileExthe excitonic transiton from S1to Sn. The insets in (b) and (c) compare the normalized dynamics for excitons (red curve) and polaron pairs (black curve) on a time scale of 20 ps. Figure 3a–c reports the Δ T / T spectra for the co-polymers PCPDT-BDT, PCPDT-BT and PCPDT-2TTP, respectively. The spectral interval reported here considers the photoinduced transition due to excitons Ex (S 1 →S n ) and the P 2 band for the co-polymers in panel b and c. The different pump-probe delays in each measurement are reported as legends together with the error bars in the Δ T / T amplitudes obtained averaging several experiments. The most important observation from these data is that the Ex band has a faster decay with respect to the P 2 bands. The absence of a distinguishable Ex band for the PCPDT-BDT polymer precludes any comparison for this material. Figure 3: Exciton and polaron pair dynamics. Δ T / T spectra recorded at different pump-probe delay times for the co-polymers PCPDT-BDT ( a ), PCPDT-BT ( b ) and PCPDT-2TTP ( c ). P 1 and P 2 indicate the polaron transitions, while Ex the excitonic transiton from S 1 to Sn. The insets in ( b ) and ( c ) compare the normalized dynamics for excitons (red curve) and polaron pairs (black curve) on a time scale of 20 ps. Full size image Another important aspect is that the Ex band does not show spectral dynamics with time, that is, it does not evolve towards the polaron features. This indicates that Ex and polaron pairs have different and uncorrelated dynamics. To further elucidate the differences between the exciton and the polaron pairs dynamics in the two co-polymers with a clear exciton photoinduced transition, we plot in the respective insets the decays on a normalized logarithmic scale. For both polymers, the Ex transition decays faster showing a clear difference in the nature of these two spectral features. The faster decay of excitons with respect to polaron pairs has been already reported by Sheng et al . [36] in homopolymers. We therefore conclude that a faster decay for hot excitons with respect to polaron pairs is a general behaviour in π-conjugated macromolecules and is probably related to the lower electron-hole overlap in polaron pairs with respect to excitons. We conclude that within the time resolution of our experiments (~150 fs), excitons and polaron pairs are formed at zero pump-probe delay and result in two populations with uncorrelated decay dynamics. Hole and electron polarons While it is commonly accepted that hole and electron polarons have similar if not identical absorption spectra in homopolymers [31] , [37] , this might not hold true in co-polymers. 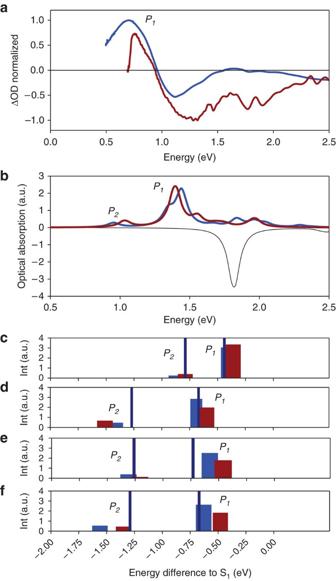Figure 4: Hole and electron polaron spectra. (a) Hole polaron spectrum (blue) obtained from the experiments ofFig. 2and electron polaron spectrum (red) obtained from charge modulation spectroscopy performed on a electron-only device with PCPDT-BDT sandwiched between an oxidized aluminium and Ca/Al electrodes. (b) Computed absorption spectrum for the neutral ground state (black, shown on the negative side of the vertical scale) and the positive (blue) and negative (red) polarons (positive sides of the vertical scale) of a PCPDT-BDT 4 units oligomer. (c,d,e,f)P1andP2absorption band intensity and relative energy positions (with respect toS1exciton energy taken as origin) for the two charged states of PCPDT-BDT, PCPDT-BT, PCPDT-2TTP and PCPDT-2TBT, respectively. The intensity of the blue (red) bars for holes (electrons) corresponds to the combined oscillator strengths for transitions located in a close (~0.2 eV) vicinity toP1andP2and their position is the corresponding intensity-weighted energy. The narrow dark blue lines indicate the experimentalP1andP2bands for positive polarons (with respect to S1energy), a lower estimation of the FWHM of the experimental polaron bands is 0.3 eV. Figure 4a shows the hole polaron spectrum from Fig. 2i , superimposed to one of the electron polaron measured by means of charge modulation spectroscopy on an electron-only diode of PCPDT-BDT (refer Methods section for device description). While the spectrum is limited by the detector sensitivity in the NIR, cutoff at 1,700 nm (0.73 eV), the two curves show very similar features suggesting that also in donor–acceptor co-polymers hole and electron polaronic transitions might exhibit similar if not identical characteristics. We were not able to obtain reliable electron-only devices from the other co-polymers. This might be due to charge injection problems. PCPDT-BDT, having the lowest electronic gap among the series presented here, is probably the only polymer with a low injection barrier between the calcium electrode used in the diodes and the LUMO. Figure 4: Hole and electron polaron spectra. ( a ) Hole polaron spectrum (blue) obtained from the experiments of Fig. 2 and electron polaron spectrum (red) obtained from charge modulation spectroscopy performed on a electron-only device with PCPDT-BDT sandwiched between an oxidized aluminium and Ca/Al electrodes. ( b ) Computed absorption spectrum for the neutral ground state (black, shown on the negative side of the vertical scale) and the positive (blue) and negative (red) polarons (positive sides of the vertical scale) of a PCPDT-BDT 4 units oligomer. ( c , d , e , f ) P 1 and P 2 absorption band intensity and relative energy positions (with respect to S 1 exciton energy taken as origin) for the two charged states of PCPDT-BDT, PCPDT-BT, PCPDT-2TTP and PCPDT-2TBT, respectively. The intensity of the blue (red) bars for holes (electrons) corresponds to the combined oscillator strengths for transitions located in a close (~0.2 eV) vicinity to P 1 and P 2 and their position is the corresponding intensity-weighted energy. The narrow dark blue lines indicate the experimental P 1 and P 2 bands for positive polarons (with respect to S 1 energy), a lower estimation of the FWHM of the experimental polaron bands is 0.3 eV. Full size image To further support the statement that hole and electron polarons have similar optical characteristics, we have performed quantum-chemical calculations and report in Fig. 4b , the hole and electron polaron spectra for a four-repeat unit oligomer of PCPDT-BDT. Interestingly, not only the calculated spectra match the experimental values for P 1 , when referenced to the theoretical position of the ground-state absorption, but also the intensity of the bands for the negatively and positively charged oligomers show very small differences. In a nutshell, this arises because both P 1 and P 2 absorption bands involve electronic transitions between delocalized molecular orbitals and 'polaronic' orbitals that owing to electronic and geometric relaxation effects self-localize over the PCPDT (BDT) units for a positive (negative) excess charge. As the polaronic wavefunction is confined spatially over segments of similar size, being either PCPDT for hole or BDT for electron, the resulting absorption spectra are similar. We next extended the calculations for the other co-polymers ( Fig. 4c–f ). The results for spectral position and relative intensities are consistent with those obtained for PCPDT-BDT, namely limited differences between cations and anions with overlapped spectral regions within the full width at half maximum (FWHM) of the experimental polaron bands (0.3 eV). Yet we note that in going from the positive to the negative polaron of the PCPDT-2TTP and -2TBT co-polymers, the main optical transitions weaken and are slightly shifted. In line with the interpretation proposed above for PCPDT-BDT, such a deviation from electron-hole symmetry in the second category of polymers arises from spreading of the PCPDT donor wavefunction over the neighbouring thiophene rings (spacers). A similar yet weaker effect occurs in PCPDT-BT and is attributed to a 'leakage' of the excess positive charge from the PCPDT to the neighbouring BT units (while this is prevented in PCPDT-BDT owing to the larger energy mismatch between frontier energy levels). Further details on calculations and polaron spectra can be found in Supplementary Figs S3 and S4 . Polaron pair yield Because of a possible partial overlap between excitonic and polaronic transitions in the ΔOD spectra of Fig. 2, we have opted for quantitatively probing the polaron pair formation considering the P -band energetically more separated from Ex , as indicated by the red vertical lines in Fig. 2i–l , and further far from the optical gap of the polymers. A quantitative estimation of the polaron pair yield on photoexcitation can be obtained by scaling the ΔOD signals at zero time delay for the number of absorbed photons in the samples. In addition, knowing the polaron absorption cross-section for the hole polaron bands and considering eventual relative differences in the contribution of electrons and holes from Fig. 4c–f , we can estimate the density of polaron pairs as detailed in the Supplementary Methods and Tables S1, S2 . 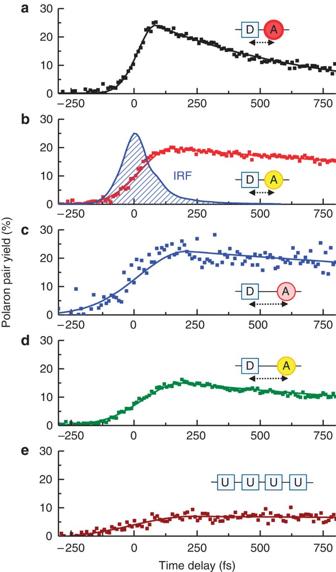Figure 5: Polaron pair generation and recombination dynamics. Time-resolved polaron pair generation after photoexcitation for the co-polymers: (a) PCPDT-BDT, (b) PCPDT-BT, (c) PCPDT-2TTP, (d) PCPDT-2TBT and (e) the homopolymer P3HT. The polaron pair generation yields areη=(24±1)%, (20±1)%, (23±2)%, (15±1.5)% and (8±2)% for PCPDT-BDT, PCPDT-BT, PCPDT-2TTP, PCPDT-2TBT and P3HT, respectively. The respective pump and probe photon energies are indicated inFig. 2. The pump photon energy for P3HT is 3.1 eV. The insets illustrate the variations in the polymer repeat units in terms of donor acceptor centre of mass distance (arrows) and acceptor strength (colour coded yellow to red). The inset inbshow the pump-probe instrument response function (IRF) for 1.55 eV (800 nm) pump and 0.41 eV (3,000 nm) probe. Solid lines are fit to the data points which are shown as squares. Figure 5 shows the rise and decay of the polaron pair density normalized by the number of photoexcitations, that is, yield (%). Low-bandgap co-polymers with acceptors having large electron affinities such as PCPDT-BDT and PCPDT-2TTP ( Fig. 5a,c ), exhibit the largest probability of polaron pair generation after photoexcitation. In contrast, PCPDT-BT and PCPDT-2TBT exhibit smaller yields modulated by the spatial separation between the donor and acceptor centre of mass. In all cases, the rise time follows the response time of our set-up at the different pump and probe wavelengths. Interestingly, also the dynamics of the recombination process differs and can be addressed to the two categories. Polymers with thiophene spacers exhibit a longer initial recombination time of the order of 5.9 and 8.8 ps for PCPDT-2TTP and -2TBT, respectively. In contrast the co-polymers without spacers show a faster recombination decay of 0.6 and 2.6 ps for PCPDT-BDT and -BT, respectively. This initial decay is likely due to the on-chain geminate recombination and remarkably in our systems it can be modulated by one order of magnitude just by changing slightly the chemical structure of the polymer. To unravel the role of acceptor strength in the recombination process, we compare co-polymers within each category. Here, we note another remarkable correlation, that is, the recombination lifetime is strongly dependent on the electron affinity of the acceptor. For instance, PCPDT-2TTP and PCPDT-BDT show faster recombination times compared with PCPDT-2TBT and PCPDT-BT, respectively. Figure 5: Polaron pair generation and recombination dynamics. Time-resolved polaron pair generation after photoexcitation for the co-polymers: ( a ) PCPDT-BDT, ( b ) PCPDT-BT, ( c ) PCPDT-2TTP, ( d ) PCPDT-2TBT and ( e ) the homopolymer P3HT. The polaron pair generation yields are η =(24±1)%, (20±1)%, (23±2)%, (15±1.5)% and (8±2)% for PCPDT-BDT, PCPDT-BT, PCPDT-2TTP, PCPDT-2TBT and P3HT, respectively. The respective pump and probe photon energies are indicated in Fig. 2 . The pump photon energy for P3HT is 3.1 eV. The insets illustrate the variations in the polymer repeat units in terms of donor acceptor centre of mass distance (arrows) and acceptor strength (colour coded yellow to red). The inset in b show the pump-probe instrument response function (IRF) for 1.55 eV (800 nm) pump and 0.41 eV (3,000 nm) probe. Solid lines are fit to the data points which are shown as squares. Full size image To place these results in the context of charge generation in organic photovoltaics, we compare the co-polymers with the response of the widely used and technologically relevant P3HT. The signal from polaron pairs in P3HT ( Fig. 5e ), monitored at 0.41 eV (ref. 30 ), exhibits the lowest yield among the materials presented here. It is gratifying to note that the yield we report, η =8±2 %, is comparable to values obtained by means of complementary techniques [38] , [39] . This last comparison supports the reasoning that donor and acceptor moieties within the polymer backbone are promoting charge separation and polaron pair formation, whereas in homopolymers, such as P3HT, charge separation is less probable and eventually driven by the energetic disorder between the polymer chromophores [40] . In the limit of the time resolution of our experiments, the primary photoexcitations are considered to be both excitons and polaron pairs. The two species are clearly distinct, as they show different dynamics ( Fig. 3 ) with excitons, which are spectrally separated from the measured ( Fig. 2i–l ) and predicted polaronic states ( Fig. 4c–f ). This is consistent with the picture drawn from previous studies on homopolymers [13] , [36] . A more exact statement on the nature of the primary photoexcitations, that is, whether excitons decay into polaron pairs or the latter are the primary photoexcitations, would require a time resolution well below 100 fs from the visible to mid-infrared. The distribution of the initial photoexcitations between these two species depends on the electronic structure of the polymer and eventually the chain conformation in the solid state [30] . Effects of chain conformation and mesoscopic morphology typically have a strong influence on the delayed formation of interchain polaron pairs [30] . On light absorption, a chromophore in the polymer chain is excited resulting in a photoexcitation with Coulomb-bound electron-hole pair, delocalized over several repeat units [41] . Such a neutral photoexcitation is expected to ionize more efficiently into localized polaron pairs if it can experience sites with imbalanced electronegativity, otherwise it localizes as an exciton. In donor–acceptor-conjugated co-polymers, sites with different electron affinity are distributed in an alternating motif along the whole polymer chain and potentially each one can act as a localization site for an electron or a hole. Such a process requires dephasing of the initial exciton and asymmetric charge localization. Thus, a large difference in electron affinity between the donor and acceptor allows for obtaining low bandgaps, as discussed in Fig. 2b–e , and enhances the formation yield of polaron pairs in co-polymers. This is valid for PCPDT-BDT and PCPDT-2TTP, with differences in η within our estimation errors. Noticeable changes in yield of about a factor of 1.3 are rather observed when comparing co-polymers with the same acceptor and with/without the spacers. PCPDT-BT and PCPDT-2TBT have virtually the same donor and acceptor and essentially differ by the thiophene spacers. PCPDT-BT shows a polaron pair yield of (20±1)%, whereas PCPDT-2TBT shows (15±1.5)%. This observation indicates that the close arrangement of donor and acceptor is important for separating the initial photoexcitation, most likely due to a larger probability of the initial exciton to experience a localizing site. Donor–acceptor co-polymers with closely spaced moieties suffer from fast recombination of the pairs. This recombination is likely due to the close average separation of the correlated geminate pairs. Interestingly, our measurements point to a beneficial role of more extended structures, such as those containing thiophene spacers, in increasing the recombination lifetime ( Fig. 5c,d ). Here, the increased spatial separation may hinder the electron hole overlap necessary for polaron pair recombination. In addition, an increased separation corresponds to a weaker Coulomb attraction and a more probable escape from the electrostatic potential by intrachain and possibly interchain thermally activated hopping. Here, we note that the delocalization of one of the carriers, in particular holes, is crucial to avoid fast recombination and seems to be an interesting approach for polaron wavefunction engineering. We also observe a trend between the electron affinity of the acceptor and the recombination lifetime within one topological category. In particular, we note that the higher the electron affinity of the acceptor, the faster the recombination time. We interpret this observation considering that the electron constituting the polaron pair might be more localized on a strong acceptor, because of the energetically deeper LUMO acceptor . In fact, polaron pair formation is expected to break the symmetry in the π-band scheme of Fig. 1a , with the electron localizing on a orbital reminiscent of the isolated acceptor LUMO [29] . On the basis of this picture, electrons in PCPDT-BDT and PCPDT-2TTP may have poor intrachain carrier mobilities, compared with co-polymers of the same category, where the LUMO acceptor is at higher energy. The recombination dynamics in P3HT support our arguments. This polymer shows the longest polaron pair decay (>12 ps) among the studied samples. Here, polaron pair formation is driven by exciton delocalization at sites with energetic disorder (typically >50 meV) [42] . A recent work by Reid et al . [43] shows that the polaron yield in P3HT depends on the degree of crystallinity because the charge separation might occur at the interface between the crystalline and amorphous regions. A less pronounced carrier localization in one of the two regions can lead to large intrachain mobilities [39] and a longer polaron pair lifetime. Our results have immediate implications for organic photovoltaics. In photovoltaic devices, the long-living charge separation is accomplished by exciton dissociation at the interface between phase-separated domains, where electrons and holes can diffuse away. Conjugated co-polymers with high yields in the formation of polaron pairs are expected to require fullerene acceptors with smaller LUMO energy offsets, as polaron pairs have a lower binding energy when compared with excitons [15] , [44] . The preference for co-polymers with either long-living polaron pairs or large generation yields may depend on the peculiar morphology of the blends with the fullerene. We envisage that blend systems with small polymer domains will be ideal for co-polymers with high yields of formation. In this configuration, polaron pairs will be separated in free charges within their lifetime, as they will be likely generated directly at the interface or close to it. For large polymer domains (>20 nm), a longer lifetime of the polaron pairs will be beneficial to favour diffusion to the interface or dissociation into free carriers followed by percolation in the most favourable phase for transport. In conclusion, we report important correlations on how the chemical structure of co-polymers is influencing the yield of generation and the recombination dynamics of polaron pairs. The generation yield seems to depend on the electron affinity of the acceptor moiety, but also shows differences when the centres of mass of similar donor and acceptor are separated. Closely spaced donor–acceptor systems suffer from a fast recombination occurring in a few picoseconds. The results provide useful input into the understanding of structure–property relationships in low-bandgap polymers for photovoltaics. Polymer synthesis and sample preparation The synthesis of the copolymer PCPDT-BT was accomplished following a procedure described in Zhu et al . [45] PCPDT-2TBT synthesis has been reported by us in Moule et al . [46] The acceptor monomers BDT and 2TTP for PCPDT-BDT and PCPDT-2TTP have been reported in Kitamura et al . [27] and Kenning et al . [47] , respectively. Synthesis of PCPDT-2TTP was carried out according to Zhou et al . [48] , while the generation of PCPDT-BDT was carried out by following Bundgaard and Krebs [49] . RR-P3HT was purchased from Aldrich. SbCl 5 was obtained from Aldrich in a glass flask and handled in a nitrogen-filled glovebox. Stille-type cross-coupling polycondensations followed by subsequent solvent-extraction steps for removing low molecular weight by-products have been used to generate and isolate the donor–acceptor co-polymers with mean number and weight average molecular weights Mn/Mw of 19,000/26,000 g mol −1 (PCPDT-BT), 6,000/13,000 g mol −1 (PCPDT-2TBT), 8,100/16,500 g mol −1 (PCPDT-BDT) and 12,500/21,400 g mol −1 (PCPDT-2TTP). All monomers and co-polymers have been characterized by 1 H and 13 C NMR spectroscopy. Solutions of the polymers in toluene with concentrations ranging from 5 to 20 mg ml −1 (according to the solubility) were spin coated at 1,000 r.p.m. for 2 min in a nitrogen-filled glovebox to obtain smooth homogeneous films on CaF 2 substrates. For the chemical doping measurements, the polymers were dissolved in 1,2-dichlorobenzene at a concentration of 15 μg ml −1 . Electron-only devices with diode structures were prepared by depositing a thin layer (30 nm) of aluminium on quartz substrates and oxidize it in air. Subsequently, the substrates were introduced in the glovebox for depositing the co-polymers from the same solutions described above. The diodes structures were completed by evaporating calcium (5 nm) and aluminium (100 nm) on top of the polymer. Doping experiments To extract the polaron cross-sections, the co-polymers in solution were doped with SbCl 5 at different concentrations as detailed in the Supplementary Figs S1, S2 and Supplementary Table S1 . Because of the high reactivity of SbCl 5 , it was stored and handled in a nitrogen-filled glovebox. In the doped solutions containing the copolymer and SbCl 5 , infrared absorption from the solvent above 3,000 nm and of the fused silica cells from 2,560 to 2,860 nm limited the probed spectral range as shown by the interrupted curves of Fig. 2i–l . Optical and charge modulation spectroscopy Absorption measurements for the thin films and the doped solutions in fused silica cuvettes were performed with an absorption spectrometer covering the spectral range from 175 to 3,300 nm. The optical density of the films at the pump wavelength was kept between 0.04 and 0.18. Time-resolved transient absorption spectra were measured with a home-built pump-probe set-up. The set-up is based on a Ti:sapphire regenerative amplifier (RegA 9060, Coherent), emitting 60 fs pulses (FWHM) with a pulse energy of 6 μJ at a central wavelength of 800 nm and a repetition rate of 90 kHz. In all, 10% of the pulse energy is used as pump pulse in the experiment by means of a beam splitter, either at the fundamental wavelength or frequency doubled to 400 nm. The pump energy density for the measurements was adjusted between 7.5 and 45 μJ cm −2 , according to the film optical density and focused to a spot diameter of ~200 μm. To keep the excitation photon density constant and comparable, twice the pump energy density was chosen when exciting at 400 nm (for P3HT). The remaining 90% of the pulse energy is used to seed an infrared optical parametric amplifier (OPA) to obtain pulses of ~100 fs duration, tunable from 0.97 to 5 μm (ref. 50 ). Careful dispersion management using the bulk dispersion of Si, Ge (positive group delay dispersion) and CaF 2 (negative) allowed for compensating the chirp originating from propagation through dispersive elements in the OPA and set-up. This resulted in a time resolution of less than 150 fs for 800 nm pump and 3 μm probe, corresponding to the cross-correlation of 130 fs (FWHM) shown in Fig. 4b . The probe spot diameter at the sample was set to half of the pump spot with a diameter of ~90 μm. The experiments for the copolymer PCPDT-2TBT (660 nm pump, 900 nm probe) were performed with a visible OPA (Coherent OPA-9450) delivering pulses with >120 fs FWHM and limiting the resolution of these experiments. Detection of the transmitted probe pulses was obtained with a liquid-nitrogen-cooled HgCdTe diode (MCT-5-N, InfraRed Associates), whose photocurrent was read out by two Lock-In Amplifiers (Standford Research) referenced to the laser repetition rate (90 kHz) and the sum frequency (96 kHz) of the repetition rate and chopping frequency (6 kHz), obtained by mechanically chopping the pump pulses. During the measurements, the films were kept under vacuum of 5×10 −6 mbar to prevent degradation processes. Charge modulation spectroscopy experiments were performed on diode structures prepared as described above. Light from a Tungsten-halogen lamp is dispersed by a spectrometer with NIR-enhanced reflectivity gratings and focused on the back contact of the diode structures. The collected light is refocused on an InGaAs photodetector referenced to the pulsing frequency of the external electronic circuit driving the charge modulation in the organic diode. To inject electrons into the diode structures, a pulse generator delivering pulses of adjustable voltage (from 2 to 10 V) and repetition rate (10–630 Hz) was connected to the diodes kept under nitrogen atmosphere. The frequency reference signal from the pulse generator was fed into the lock-in amplifier detecting the signal from the photodiode. For each set of samples, optimal values for voltage and frequency were tested. Quantum-chemical modelling The ground-state geometry of oligomers of increasing size (up to four repeating units) has first been optimized at the Hartree–Fock semi-empirical Austin Model 1 (AM1) level for the neutral molecules and by combining AM1 with a configuration interaction scheme for the charged molecules [33] . To allow for direct comparison between the different polymers, we focused on chains of similar physical lengths, namely featuring four repeating units for PCPDT-BDT and PCPDT-BT and three units in the case of PCPDT-2TTP and PCPDT-2TBT. These oligomers seem to be long enough to mimic the photo-physical behaviour of the corresponding polymers. In all calculations, the ethyl-hexyl chains have been replaced by hydrogen atoms, as they are not participating to the description of the lowest optical absorption bands. The absorption spectra have been simulated on the basis of the electronic excited states obtained by coupling the AM1 model to a full configuration interaction scheme involving 20 occupied and 20 unoccupied energy levels. How to cite this article: Tautz, R. et al . Structural correlations in the generation of polaron pairs in low-bandgap polymers for photovoltaics. Nat. Commun. 3:970 doi: 10.1038/ncomms1967 (2012).